Room temperature ferromagnetism in Teflon due to carbon dangling bonds The ferromagnetism in many carbon nanostructures is attributed to carbon dangling bonds or vacancies. This provides opportunities to develop new functional materials, such as molecular and polymeric ferromagnets and organic spintronic materials, without magnetic elements (for example, 3 d and 4 f metals). Here we report the observation of room temperature ferromagnetism in Teflon tape (polytetrafluoroethylene) subjected to simple mechanical stretching, cutting or heating. First-principles calculations indicate that the room temperature ferromagnetism originates from carbon dangling bonds and strong ferromagnetic coupling between them. Room temperature ferromagnetism has also been successfully realized in another polymer, polyethylene, through cutting and stretching. Our findings suggest that ferromagnetism due to networks of carbon dangling bonds can arise in polymers and carbon-based molecular materials. Ferromagnets and their applications have been widely studied and explored for several decades. Classic ferromagnetic materials typically contain magnetic elements, such as Fe, Co, Ni or rare earth elements with partially filled d or f orbitals. Recently, intensive attention has been drawn to ferromagnetism (FM) in 'non-magnetic' materials, such as carbon-based systems [1] , [2] , [3] . Investigations of FM in various carbon nanostructures have revealed that ferromagnetic coupling in such systems originates from intrinsic structural defects, such as dangling bonds [4] , [5] and vacancies [2] , [6] , which can change the localized electronic states at Fermi energy and eventually lead to a stable magnetic ordering. Curie temperature obtained for these C nanostructures is generally high, for example, 1,000±100 K for carbon nanotubes [7] , 460 K for graphite [8] and 764 K in the case of graphene [9] . FM was also reported in polyimide film after heat treatment [10] , which is believed to be associated with structural defects. Molecular and polymeric ferromagnets have been intensively studied in the past three decades [4] , [11] , [12] , [13] , [14] , [15] . Usually, transition metal elements are introduced into molecular compounds to induce FM. The FM due to C dangling bonds/defects in C nanostructures opens new opportunities, as C chain structure is the backbone in many polymeric and molecular materials. In this work, we demonstrate that room temperature FM can be realized in Teflon through very simple methods—cutting or mechanical stretching. Teflon is chosen because of its good chemical stability, high melting temperature and availability in the form of thin and uniform tape, which can be easily cut or stretched. The FM in Teflon is originated from carbon dangling bonds. Our first-principles calculations revealed a strong ferromagnetic coupling when the C dangling bonds form a two-dimensional (2D) or quasi-2D network. 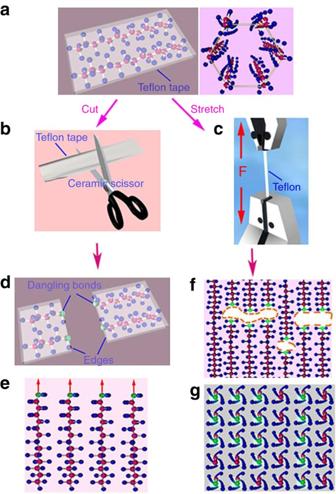Figure 1: Experimental procedure. (a) Schematic illustration of carbon chain structure in Teflon tape (left) and hexagonal arrangement of carbon chains in Teflon (right). Carbon and fluorine atoms are shown in red and blue, respectively. (b) Illustration of cutting of a Teflon tape using a pair of ceramic scissors. (c) Illustration of stretching of a Teflon tape. (d) Schematic illustration of dangling bonds created after cutting. (e) Schematic illustration (side view) of ferromagnetic ordering formed in the 2D network of carbon dangling bonds. Under-coordinated carbon atoms (with a dangling bond) are shown in green. The red arrows indicate magnetic moments. (f) A schematic illustration (side view) of C dangling bonds formed in Teflon by mechanical stretching. C dangling bonds are highly concentrated on the surface of nano-sized voids generated by the mechanical stretching. (g) A cross-sectional view (top view) of 2D network of C dangling bonds in crystalline Teflon subjected to mechanical stretching. Carbon atoms with and without dangling bonds are shown in green and red, respectively. Structural and compositional examinations Figure 1 presents a schematic view of our experiments, and illustrates how cutting or stretching of the Teflon tape can lead to a network of C dangling bonds. A thin and high-purity Teflon tape with a pseudo-hexagonal structure ( Fig. 1a ) is subjected to cutting ( Fig. 1b ) or stretching ( Fig. 1c ). After the cutting, a 2D network of C dangling bonds can be formed in the cross-section of the broken Teflon tape. Each C dangling bond carries a magnetic moment of 1 μ B and the C dangling bonds in the 2D network are ferromagnetically coupled, as shown in Fig. 1d,e . Following a mechanical stretching with a large strain, a network of C dangling bonds may be generated. Figure 1f,g illustrates a possible distribution of C dangling bonds, which are largely concentrated on the surface of strain-induced voids and are ferromagnetically coupled. Figure 1: Experimental procedure. ( a ) Schematic illustration of carbon chain structure in Teflon tape (left) and hexagonal arrangement of carbon chains in Teflon (right). Carbon and fluorine atoms are shown in red and blue, respectively. ( b ) Illustration of cutting of a Teflon tape using a pair of ceramic scissors. ( c ) Illustration of stretching of a Teflon tape. ( d ) Schematic illustration of dangling bonds created after cutting. ( e ) Schematic illustration (side view) of ferromagnetic ordering formed in the 2D network of carbon dangling bonds. Under-coordinated carbon atoms (with a dangling bond) are shown in green. The red arrows indicate magnetic moments. ( f ) A schematic illustration (side view) of C dangling bonds formed in Teflon by mechanical stretching. C dangling bonds are highly concentrated on the surface of nano-sized voids generated by the mechanical stretching. ( g ) A cross-sectional view (top view) of 2D network of C dangling bonds in crystalline Teflon subjected to mechanical stretching. Carbon atoms with and without dangling bonds are shown in green and red, respectively. Full size image An X-ray diffraction (XRD) study of the Teflon tape showed a crystalline pseudo-hexagonal structure with a = b =5.66 Å and c =19.5 Å, similar to the values reported by Bunn and Howells [16] . Raman spectroscopy analysis showed spectral features of crystalline Teflon. It is noted that annealing and mechanical stretching do not result in any noticeable changes in the XRD and Raman spectra ( Supplementary Fig. S1 ). Energy dispersive X-ray spectroscopy (EDS) and X-ray photoelectron spectroscopy (XPS) showed that only fluorine (F) and carbon (C) were present in the sample ( Supplementary Fig. S1 ). All the peaks in Raman spectra could be well identified with modes of crystalline Teflon [17] , [18] . There is no detection of other elements (particularly 3 d elements), as analysed by XPS, secondary ion mass spectrometry (SIMS) and inductively coupled plasma (ICP) measurements under the maximum detection limit of 1 p.p.m. As contamination of magnetic elements is a common source of the observed FM in non-magnetic materials, it is important to rule out such possibility. At the detection limit of 1 p.p.m., contamination of Fe, which has the highest magnetization among the 3 d elements, would result in a saturation magnetization ( M s ) of 0.2 memu g −1 . As this value is much smaller than the measured magnetization of our samples, we conclude that the FM in the Teflon sample is not due to contamination by magnetic elements. In addition, as discussed below, the magnetization in Teflon can be switched 'on' and 'off' through alternating annealing under Ar and H 2 O atmospheres, which further confirms that the observed FM in our samples is intrinsic. Mechanical stretching and cutting We started our experiment with mechanical stretching of Teflon tape in air with a tensile test machine. A typical force-strain plot of the stretching process is depicted in Fig. 2a . Necking starts at a strain of ∼ 35% (corresponding to a stress of ∼ 10 MPa) and the Teflon tape is completely broken at a strain of around 100%. The Teflon tape exhibited diamagnetic as shown in Fig. 2b . After the mechanical stretching until broken down, the magnetization curve showed a mixture of ferromagnetic and diamagnetic signals, as shown in Fig. 2c . Magnetic measurements of the original Teflon tape and tapes after mechanical stretching (with different mechanical strains) were carried out at room temperature and the results are shown in Fig. 2d (after the substation of the diamagnetic signal). From the M–H loops, it is clear that the original Teflon tape (as-received) is non-magnetic. However, after subjecting to a strain of 30–40%, the M–H curves show a characteristic hysteresis loop and the saturation magnetization increases with increasing mechanical strain. The saturation magnetization reaches its maximum value of ∼ 0.3 memu g −1 when the Teflon tape is broken. The coercivity in the order of 100 Oe is clearly observed in the M–H loop, indicating FM in the samples. The threshold strain for emerging FM coincides with the necking of the Teflon tape (strain ∼ 35%), suggesting that the FM in the Teflon tape is related to its structural deformation. 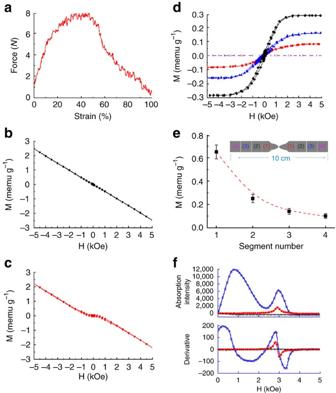Figure 2: Tuning of magnetic properties of Teflon tape by mechanical stretching. (a) Force–strain curve of Teflon tape subjected to mechanical stretch. (b) M–H loop of the original Teflon tape (without stretch). The Teflon tape has a diamagnetic signal. (c) Teflon subjected to mechanical stretch until broken down. No background subtraction has been performed. The ferromagnetic signal is mixed together with the diamagnetic signal. After appropriate correction for the diamagnetic background at high fields, the hysteresis loops were obtained as shown ind. (d) Magnetization curves of as-received Teflon tape (unstretched) and tapes subjected to different strains after the subtraction of the diamagnetic signal (unstretched (violet); 35% strain (red); 60% strain (blue); 100% strain (black)). (e) Measured saturation magnetization in different segments of a stretched Teflon tape from necking point (Segment 1) to the unstretched end of the tape (Segment 4). The typical length and mass of Teflon tapes used in the experiment are 10 cm and 0.08 g, respectively. Each error bar was calculated based on measurements of three samples. (f) Electron spin resonance (ESR) spectroscopy of Teflon tapes under different strains: unstretched and non-magnetic tape (black), Segment 1 (blue) and Segment 4 (red). Segments 1 and 4 are shown inFig. 1e. Figure 2: Tuning of magnetic properties of Teflon tape by mechanical stretching. ( a ) Force–strain curve of Teflon tape subjected to mechanical stretch. ( b ) M–H loop of the original Teflon tape (without stretch). The Teflon tape has a diamagnetic signal. ( c ) Teflon subjected to mechanical stretch until broken down. No background subtraction has been performed. The ferromagnetic signal is mixed together with the diamagnetic signal. After appropriate correction for the diamagnetic background at high fields, the hysteresis loops were obtained as shown in d . ( d ) Magnetization curves of as-received Teflon tape (unstretched) and tapes subjected to different strains after the subtraction of the diamagnetic signal (unstretched (violet); 35% strain (red); 60% strain (blue); 100% strain (black)). ( e ) Measured saturation magnetization in different segments of a stretched Teflon tape from necking point (Segment 1) to the unstretched end of the tape (Segment 4). The typical length and mass of Teflon tapes used in the experiment are 10 cm and 0.08 g, respectively. Each error bar was calculated based on measurements of three samples. ( f ) Electron spin resonance (ESR) spectroscopy of Teflon tapes under different strains: unstretched and non-magnetic tape (black), Segment 1 (blue) and Segment 4 (red). Segments 1 and 4 are shown in Fig. 1e . Full size image In order to understand the relationship between structure deformation and magnetic properties, we cut the stretched Teflon tape into four parts and labelled them as Segment 1 (near the break point, with the highest mechanical strain) to Segment 4 (the least stretched part), as shown in Fig. 2e . The measured saturation magnetization decreases from Segment 1 to Segment 4, with Segment 1 showing the highest saturation magnetization, and Segment 4 the lowest, indicating that the room temperature FM is strongly correlated to strain or structural deformation, and may be due to broken bonds (dangling bonds) in Teflon after the stretching ( Fig. 2e ). Electron spin resonance (ESR) spectroscopy was used to confirm the intrinsic FM of mechanically stretched Teflon tapes. Three samples were selected for the study, namely, as-received non-magnetic Teflon tape, stretched tape with a very weak magnetism (Segment 4) and stretched tape with strong magnetism (Segment 1). The non-magnetic tape has no signal in the derivative and absorption, indicating absence of unpaired electrons ( Fig. 2f ). Segment 4 has a paramagnetic signal, indicating presence of unpaired electrons without magnetic coupling. For Segment 1, the absorption can be considered a mixture of two parts. Besides the paramagnetic signal in the derivative curve, a broad and non-symmetric curve appears at low field, as shown in the upper panel of Fig. 2f . This peak is an indication of ferromagnetic resonance and its appearance confirms FM in the sample [19] . The paramagnetic signal observed in Segment 4 is likely due to isolated C dangling bonds, which are created at a low strain. As the mechanical strain increases, the density of C dangling bonds increases and the C dangling bonds begin to interact. The exchange coupling between the C dangling bonds in the interacting network of C dangling bonds results in a ferromagnetic state at high strain (Segment 1). The paramagnetic signal remains in Segment 1, as shown in Fig. 2f , as there are always isolated non-interacting C dangling bonds present in the sample even at a high strain. For the paramagnetic component, the g factor values estimated from Fig. 2d are 2.10 and 2.12 for Segment (1) and Segment (4), respectively, which are higher than that of free ions ( g =2.0023). The high g factor may be due to the strong anisotropy formed by stretching [20] . Cutting is another simple way to generate C dangling bonds in the Teflon tape. A 2D network of C dangling bonds can be formed in the cross-sectional plane, as illustrated in Fig. 1f . In this work, we cut the Teflon tape with a pair of ceramic blade scissors in different environments ( Table 1 ). Superconducting quantum interference device measurement indicates that the Teflon tapes cut in the air, pure N 2 , pure Ar or 0.1% H 2 /Ar are ferromagnetic at room temperature, whereas no FM was observed when Teflon tape was cut under 2.5%H 2 /Ar. This indicates that the magnetism of the Teflon is strongly dependent on the environment. As the magnetization of a single cut is too weak to be detected, all samples were prepared with 100 cuts from the same Teflon tape. The saturation magnetization of Teflon cut in air is ∼ 0.09 memu g −1 ( Table 1 ). This value is close to the expected magnetization derived based on the number of C dangling bonds in the cross-section area after cutting, if each C dangling bond carries a magnetic moment of 1 μ B and magnetic moments from various C dangling bonds are ferromagnetically coupled. The low value of saturation magnetization is because Teflon tape is very thin (in the μm range). Nevertheless, the FM in the cut Teflon samples confirms that FM in Teflon is due to the 2D network of C dangling bonds. It is interesting to note that ESR spectrum of the cut Teflon slips shows a similar ferromagnetic shape as that of the mechanically stretched Teflon tape. This suggests that the origin of FM in the cut Teflon tape and the mechanically stretched Teflon tape are same, that is, 2D network of C dangling bonds. Table 1 A summary of magnetization M s of Teflon and polyethylene after cutting. Full size table Heat treatment Stability of the FM is important for potential engineering applications. To examine how the annealing temperature and atmosphere affect the stability of FM, we first annealed Teflon tapes (stretched and as-purchased) under different atmospheres, and found surprisingly that the saturation magnetization of the mechanically stretched Teflon tape increased from 0.3 memu g −1 (as shown in Fig. 2e ) to 1–3 memu g −1 after annealing at 100–200 °C for 2 h in Ar atmosphere. In addition, the as-purchased (unstretched) non-magnetic Teflon tape also became ferromagnetic after annealing at 100–200 °C in Ar atmosphere, with saturation magnetization of 1–3 memu g −1 at room temperature. This motivated us to carry out a systematic study to investigate the effects of annealing temperature and atmosphere on the FM of the as-purchased non-magnetic Teflon tapes. 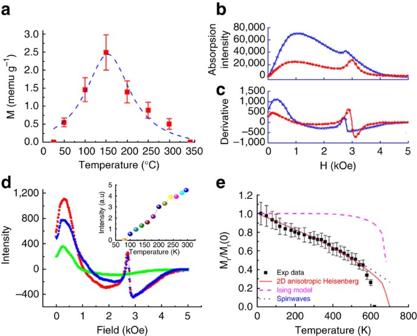Figure 3: Effects of annealing temperature under Ar atmosphere on magnetic properties of Teflon tape. (a) Saturation magnetizationMsas a function of annealing temperature of the Teflon tape annealed in pure Ar for 2 h (dashed blue line is a guide for the eyes). EachMsvalue was obtained from averaging of six samples. (b,c) ESR results (absorption intensity and derivative) of the two samples annealed at 50 (red) and 150 °C (blue), respectively. (d) ESR spectra taken at different temperatures (300 K (red), 180 K (blue) and 80 K (green)) for the ferromagnetic Teflon (after annealing at 150 °C). The inset shows the integrated intensity of the paramagnetic component as a function of temperature. (e) The normalized remanent magnetization as a function of temperature, and fittings to various models.Mr(0)=0.67 memu g−1. These error bars were obtained based on three measurements. Figure 3a shows the annealing temperature dependence saturation magnetization of the Teflon tape, which was annealed for 2 h in pure Ar. The magnetization increases with increasing annealing temperature until reaching a maximum of 2.5 memu g −1 at 150 °C, and then decreases with further increase in annealing temperature. A pro-longed annealing at 150 °C (up to 10 h) did not result in any significant change in the saturation magnetization. The FM eventually vanishes when the annealing temperature reaches 350 °C, which is close to the melting temperature of Teflon (340–350 °C), as determined by our differential scanning calorimetry and thermogravimetric analysis measurements ( Supplementary Fig. S2 ). From the value of saturation magnetization (2–3 memu g −1 ) of Teflon tape that was annealed in Ar for 2 h, one can derive that ∼ 0.001% of the C atoms in the Teflon sample have dangling bonds. As this concentration is beyond the detection limit of Raman, Fourier transform infrared spectroscopy (FTIR) and other structural characterization techniques, we performed ESR measurements. Figure 3b,c shows ESR results of the two samples, which are annealed at 50 °C (with a saturation magnetization M s =0.51 memu g −1 ) and 150 °C (with M s =2.5 memu g −1 ), respectively. The sample with the lower magnetization (0.51 memu g −1 ) consists of a mixture of a paramagnetic component and a ferromagnetic component. For the sample with higher magnetization (2.5 memu g −1 ), the paramagnetic signal became very weak, indicating that a relatively large quantity of C dangling bonds is present and they are ferromagnetically coupled. We estimated g -factor to be 2.03 for the sample with a weak magnetization after annealing at 50 °C and 2.21 for the sample with a stronger saturation magnetization after annealing at 150 °C. The increase in g -factor with increasing magnetization might be related with the presence of a strong ferromagnetic resonance [21] , [22] . Temperature dependence of ESR analysis ( Fig. 3d ) shows that the paramagnetic signal decreases with decreasing temperature and disappears at ∼ 80 K, indicating the possibility of a broad paramagnetism/FM transition, probably due to structural inhomogeneity (as suggested in Fig. 1f ). Figure 3: Effects of annealing temperature under Ar atmosphere on magnetic properties of Teflon tape. ( a ) Saturation magnetization M s as a function of annealing temperature of the Teflon tape annealed in pure Ar for 2 h (dashed blue line is a guide for the eyes). Each M s value was obtained from averaging of six samples. ( b , c ) ESR results (absorption intensity and derivative) of the two samples annealed at 50 (red) and 150 °C (blue), respectively. ( d ) ESR spectra taken at different temperatures (300 K (red), 180 K (blue) and 80 K (green)) for the ferromagnetic Teflon (after annealing at 150 °C). The inset shows the integrated intensity of the paramagnetic component as a function of temperature. ( e ) The normalized remanent magnetization as a function of temperature, and fittings to various models. M r (0)=0.67 memu g −1 . These error bars were obtained based on three measurements. Full size image Figure 3e shows the temperature dependence of the normalized remnant magnetization ( M r / M r (0)) for the sample annealed at 150 °C The experimental data (solid squares with error bars) can be described by the spin-wave theory based on the uniaxially anisotropic 2D Heisenberg model, in conjunction with the Ising model [8] , [23] . The blue dotted line and magenta dashed curve in Fig. 3e are derived from the spin-wave theory [24] and the Ising model [25] , respectively. The fitting parameters used here are the critical temperature of spin-wave T c sw =1,160 K, anisotropy Δ=0.001, and Curie temperature T c =680 K. At low temperature ( T <550 K), the magnetization is a linear function of temperature, which can be described by spin-wave theory based on the 2D Heisenberg model. Spin flip excitation is considered near Curie temperature and the Ising model provides a better description for spin flip excitation. It is unequivocal that the theoretical model (red curve) from the conjunction of spin-wave theory and the Ising model fit the measured data well with Curie temperature of ∼ 680 K. It should be noted that the high Curie temperature is in consistence with those reported in carbon nanostructures (that is, 1,000 K for carbon nanotubes, 764 K for graphene and 460 K for graphite) [7] , [8] , [9] . On the basis of the above discussion, the disappearance of FM at 340–350 °C (613–623 K) can be attributed to melting of Teflon. 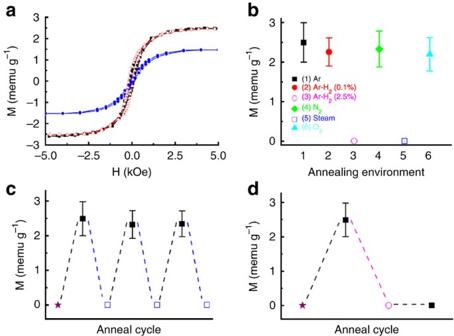Figure 4: Effects of cyclic annealing in different environments. (a) Hysteresis loops of Teflon tape after annealing in pure Ar (black), after storage in desiccator for 25 days (red) and after the exposure in air for 25 days (blue). (b) Saturation magnetization of Teflon tapes after annealing at 150 °C under different atmospheres. (c) Saturation magnetizationMsof Teflon tape subjected to alternative annealing in pure Ar (black full-square) and water steam (blue open square) at 150 °C for 2 h (the violet star represents the as-received tape). (d) Saturation magnetizationMof Teflon tape (violet star for as-received), subjected to annealing under pure Ar (black full square), subsequently annealed under 2.5% H2/Ar (magenta open circle), and again under pure Ar (black full square) at 150 °C for 2 h. Each magnetization value (M) is averaged from measurements of three samples. Figure 4a shows that the FM is stable under a dry environment (after 25 days in a desiccator). However, the saturation magnetization is reduced significantly after an air exposure for 25 days. As mentioned earlier, Teflon cut under the high partial pressure of H 2 atmosphere did not exhibit FM. To investigate how the atmosphere affects the magnetic property of the Teflon, we performed heat treatment in different atmospheres. The as-purchased Teflon tape was used as the starting material and the annealing was done at 150 °C. As shown in Fig. 4b , FM appears after annealing in pure Ar, N 2 , 0.1%H 2 /Ar or 20%O 2 /Ar, but not after annealing under water steam and 2.5%H 2 /Ar. This indicates that the FM is unstable under water steam or H 2 -containing atmosphere with a relatively high H 2 partial pressure. As the H 2 partial pressure in air is in the order of 10 −6 atm (0.0001%), and the FM is stable under 0.1%H 2 /Ar ( Fig. 4b and Table 1 ), the decrease in magnetization after a 25 day of air exposure should attribute mainly to humidity (humidity in Singapore is usually high). Figure 4: Effects of cyclic annealing in different environments. ( a ) Hysteresis loops of Teflon tape after annealing in pure Ar (black), after storage in desiccator for 25 days (red) and after the exposure in air for 25 days (blue). ( b ) Saturation magnetization of Teflon tapes after annealing at 150 °C under different atmospheres. ( c ) Saturation magnetization M s of Teflon tape subjected to alternative annealing in pure Ar (black full-square) and water steam (blue open square) at 150 °C for 2 h (the violet star represents the as-received tape). ( d ) Saturation magnetization M of Teflon tape (violet star for as-received), subjected to annealing under pure Ar (black full square), subsequently annealed under 2.5% H 2 /Ar (magenta open circle), and again under pure Ar (black full square) at 150 °C for 2 h. Each magnetization value ( M ) is averaged from measurements of three samples. Full size image To further understand the effects of water vapour or H 2 on the magnetic property of Teflon, a cyclic annealing was performed and the results are shown in Fig. 4c,d . Using the non-magnetic as-purchased Teflon tape as the starting material, the first annealing in the Ar atmosphere at 150 °C induces room temperature FM with a saturation magnetization of 2–3 memu g −1 . However, a subsequent annealing in steam at 150 °C nearly eliminates the FM. Surprisingly, annealing under Ar atmosphere at 150 °C subsequently fully recovers the FM. The ferromagnetic state can be switched 'on' and 'off' by performing cyclic annealing in Ar and steam, as shown in Fig. 4b . Presence of water molecules in Teflon tape was examined using FTIR. A weak peak was found at the wavenumber of 3,440 cm −1 in the as-purchased Teflon tape, indicating presence of adsorbed water molecules [26] , [27] . After annealing in Ar at 150 °C, the peak disappeared. But it appeared again with a similar relative intensity after subsequent treatment in steam. Figure 4d shows the annealing effect under H 2 atmosphere (2.5%H 2 -Ar). Room temperature FM appeared after first annealing of the as-purchased Teflon tape under pure Ar atmosphere at 150 °C. Similar to the steam annealing, the subsequent annealing in 2.5%H 2 -Ar led to the disappearance of FM. However, the FM cannot be recovered after a further annealing at 150 °C in pure Ar. Modelling and first-principles calculations On the basis of the above results, we might plausibly propose a mechanism for the FM based on the presence of a large quantity of C dangling bonds as a result of breaking of carbon chains because of cutting or stretching. Each of these C dangling bonds carries a magnetic moment of 1 μ B . If the mechanical strain is relatively small, the C dangling bonds are isolated and non-interacting, leading to a paramagnetic state. At a large strain, the density of C dangling bonds increases, and a strong exchange coupling between them results in a ferromagnetic state. The C dangling bonds are relatively stable in Teflon under ambient condition. However, when the Teflon tape is exposed to air for a long time, FM may vanish due to saturation of C dangling bonds by attachment of water molecules. The attachment process can be accelerated by annealing in water steam ( Fig. 4 ). However, the binding of water molecules to the C dangling bonds is relatively weak, and they can be removed by annealing in Ar. Therefore, the vanished FM in Teflon tape after steam annealing can be recovered by Ar annealing. As shown in Fig. 2 , a mechanical strain of ∼ 100% can result in magnetization up to 0.3 memu g −1 . The commercially available Teflon tape may contain a large quantity of C dangling bonds during the fabrication process (to the final thickness stage of micrometre). However, most Teflon tapes do not show FM in the as-received state, probably due to saturation of the C dangling bonds by water molecules. A simple annealing in Ar removes the water molecules and leads to room temperature FM, as demonstrated in Fig. 4 . We also took ESR spectrum of Teflon after annealing under H 2 or in water vapour. No ferromagnetic resonance was shown for these samples and their ESR spectra were the same as that of non-magnetic tape as shown in Fig. 2f . To verify this hypothesis, we examined a bulk Teflon, which should contain negligible amount of C dangling bonds as bulk Teflon is less stretched during fabrication. Interestingly, no FM could be observed in the bulk Teflon after Ar annealing at 150 °C. Furthermore, the expected FTIR peak at 3,440 cm −1 was not seen after the bulk Teflon was annealed in water steam, confirming that water molecules are not incorporated in bulk Teflon. On the other hand, the bulk Teflon becomes magnetic after cutting. These results suggest that Ar annealing does not lead to FM in bulk Teflon due to absence of dangling bonds. But cutting or stretching may generate C dangling bonds in the bulk Teflon and result in FM. The decrease in magnetization after annealing under Ar atmosphere at 200 °C or higher and the disappearance of FM near the melting temperature of Teflon ( ∼ 350 °C) can be explained by structural reconstruction, as the Teflon undergoes significant structural change above 200 °C (ref. 16 ). For example, C dangling bonds can be eliminated or reduced by joining dangling bonds together (recombination) at higher temperatures. On the other hand, C dangling bonds may be saturated by H via formation of C–H bonds under a relatively high H 2 partial pressure (in the order of 2.5 vol%), which also leads to the disappearance of FM. Unlike the attachment of H 2 O, the formation of C–H bond is nonreversible, as FM cannot be recovered after a subsequent Ar annealing at various temperatures, up to 250 °C. Reversible hydrogenation phenomenon has been observed in graphene after annealing at a temperature of 450 °C (ref. 28 ). However, for Teflon, high annealing temperature above 250 °C may cause structural damage. To understand the ferromagnetic ordering in the magnetic Teflon tape, we carried out first-principles calculations based on the density functional theory. As mentioned above, the crystalline Teflon has a pseudo-hexagonal structure consisting of helical chains. In our first-principles calculations, we first focused on magnetic ordering between two C dangling bonds and considered the head-to-head configuration of a single polytetrafluoroethylene molecule, which mimics the breaking of a single Teflon chain, as shown in Supplementary Fig. S3a . Our calculations yield an equilibrium C–C bond length of 1.56 Å with a bonding energy of 3.46 eV, which agrees well with reported values [29] . It is found that the system energetically favours a non-magnetic ground state when the C–C separation is smaller than 2.5 Å. However, at large C–C separation, a localized magnetic moment of 1 μ B per C dangling bond emerges and magnetic ordering starts to form when the C–C bond length reaches about 3 Å. The energy difference between the FM and the antiferromagnetism (AFM) states shows a positive peak at around 3 Å, indicating that the AFM state is more favourable than the FM state for the two C dangling bonds in the head-to-head configuration. Instead, the exchange coupling could be realized through the interactions between C dangling bonds in neighbouring helical chains, as shown in inset of Supplementary Fig. S3b . Our first-principles calculations show that two C dangling bonds in the parallel arrangement are also antiferromagnetically coupled with a bonding energy maximum around an inter-chain distance of 3 Å ( Supplementary Fig. S3b ) and with a coupling energy of 0.18 eV. The energy difference between FM and AFM ( E FM−AFM ) decreases rapidly to zero if the C dangling bonds are separated by more than 4 Å. It is noted that the inter-chain distance in Teflon is around 5.5 Å. Both head-to-head and parallel arrangements of two C dangling bonds are paramagnetic (no exchange coupling) at an inter-chain distance ranging from 4.5 to 6.0 Å. As a matter of fact, when a Teflon tape is cut, there should be a large concentration of C dangling bonds in the cross-sectional plane and it is highly possible that these dangling bonds form a 1D chain or a 2D network, as illustrated in Fig. 5a,b . In the case of 1D chain of C dangling bonds, our density functional theory calculations show that when the distance between the Teflon chain is around 4.8 Å, the system energetically favours a ferromagnetic state, and its total energy is 59 meV lower than that of the AFM state. This inter-chain distance is close to the polymer chain separation (around 5.5 Å) determined from our XRD measurements ( Supplementary Fig. S1 ). The magnetic coupling between C dangling bonds in the 2D network is even stronger. Our calculations revealed a ferromagnetic coupling of 82 meV, when the Teflon chains are separated by 4.9–5.0 Å ( Fig. 5b ), which is close to the expected inter-chain separation (5.0–5.5 Å) in the hexagonal crystal structure of Teflon. The ferromagnetic coupling between C dangling bonds can be clearly seen from the spin densities as shown in Fig. 5c,d . The spin-up densities are mainly localized around carbon atoms at the end of Teflon chains and they couple to each other via fluorine atoms between the carbon backbones. These spin-up densities also propagate into carbon atoms along the Teflon chains but decay rapidly. At the same time, these states are well localized in energy. The calculated total spin-polarized density of states (DOS) shows the localization of these states at the Fermi level ( Fig. 5e ) and a large splitting between the spin-up and spin-down states. Only the spin-up component is occupied, while the spin-down component is empty. 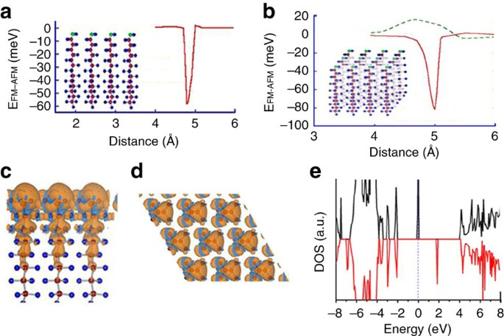Figure 5: Results of first-principles calculations and mechanism of ferromagnetism. (a) The energy difference between ferromagnetic and antiferromagnetic states (EFM–EAFM) as a function of C–C distance in the 1D chain of C dangling bonds; (b) The energy difference between ferromagnetic and antiferromagnetic states (EFM–EAFM) as a function of C–C distance in the 2D network of C dangling bonds (solid line) and in the 2D network of C dangling bonds attached with H2O (dashed line); (c) side view and (d) top view of spin density in the 2D network of C dangling bond model of Teflon tape; the spin density is defined as the difference between spin-up and spin-down electron densities. Positive spin density is shown in brown (upper) and negative (lower) ones in blue. Carbon and fluorine atoms are shown using red and blue balls, respectively. (e) Spin-polarized density of states of 2D C dangling bonds; spin-up (upper) is shown in black and spin-down (lower) in red. The Fermi energy is indicated by the vertical dashed line. All results are obtained based on a hybrid functional (PBE0). Figure 5: Results of first-principles calculations and mechanism of ferromagnetism. ( a ) The energy difference between ferromagnetic and antiferromagnetic states ( E FM – E AFM ) as a function of C–C distance in the 1D chain of C dangling bonds; ( b ) The energy difference between ferromagnetic and antiferromagnetic states ( E FM – E AFM ) as a function of C–C distance in the 2D network of C dangling bonds (solid line) and in the 2D network of C dangling bonds attached with H 2 O (dashed line); ( c ) side view and ( d ) top view of spin density in the 2D network of C dangling bond model of Teflon tape; the spin density is defined as the difference between spin-up and spin-down electron densities. Positive spin density is shown in brown (upper) and negative (lower) ones in blue. Carbon and fluorine atoms are shown using red and blue balls, respectively. ( e ) Spin-polarized density of states of 2D C dangling bonds; spin-up (upper) is shown in black and spin-down (lower) in red. The Fermi energy is indicated by the vertical dashed line. All results are obtained based on a hybrid functional (PBE0). Full size image As shown in Supplementary Table S1 , we also considered magnetic coupling of other possible configurations of C dangling bonds, and in particular when two C dangling bonds in two neighbouring parallel Teflon chains are not in the same cross-sectional plane. This could occur when the Teflon tape is subjected to a tensile stress. Results of our calculations show that the ferromagnetic coupling decreases rapidly with the separation of the C dangling bonds in the direction of the Teflon chains. When the two C dangling bonds are separated by one C–C unit (2.62 Å) along the direction of the Teflon chain (Model 6 in Supplementary Table S1 ), FM remains but with a much reduced exchange-coupling energy (41 meV). When the C dangling bonds are separated by two C–C units (5.24 Å) or more, the system becomes paramagnetic (Model 7 in Supplementary Table S1 ). These results, together with the non-ferromagnetic coupling between two C dangling bonds in the head-to-head configuration ( Supplementary Fig. S3 ), suggest that even though strain may generate a 3D network of C dangling bonds when the Teflon tape is subjected to mechanical stretching, ferromagnetic coupling occurs mainly between C dangling bonds in plane perpendicular to the strain direction or in strain-induced lateral voids (as illustrated in Fig. 1f ). As such voids are mainly concentrated near the breaking point of the Teflon tape, the FM decreases rapidly away from the breaking point, as shown in Fig. 2e . As the ferromagnetic coupling is mainly between C dangling bonds in neighbouring Teflon chains, and it is relatively difficult to change the configurations for C dangling bonds from neighbouring Teflon chains to form a covalent bond, the FM in Teflon is relatively stable. Based on our experimental results, structural reconstruction may take place at temperature above 200 °C, which is in good agreement with results of Bunn et al . [22] However, our experimental results indicate that the FM in Teflon is unstable when the samples are exposed to air. The adsorption of water molecules or formation of bonds between the under-coordinated C and H or OH is likely the reason for the elimination of FM. Results of our first-principles calculations confirm that a strong bond can be formed between the under-coordinated C and H or OH. The bonding energy can be 4.5–5.0 eV ( Supplementary Table S2 ). Once the C dangling bonds are saturated by H or OH, they cannot be removed, which explains the experimental results that the formation of C–H bond under a high H 2 partial pressure annealing eliminates FM permanently ( Fig. 4d ). However, the vanished FM after steam annealing can be recovered. Therefore, the elimination of FM by steam annealing cannot be due to formation of bonds between the under-coordinated C and H or OH. To clarify this issue, we performed further calculations to examine the possible attachment of water molecules to the C dangling bonds as well as the possible magnetic ordering. It is found that a stable structure with formation energy of −0.48 eV can be formed when the H ions of the water molecule face the F ions and the O ion is next to the under-coordinated C atom, as shown in Fig. 5b . Results of our calculations also show that the energy difference between ferromagnetic and AFM states in this structure is greatly reduced and a weak AFM is favourable, as shown in Fig. 5b . The states of dangling bonds are very localized and higher in energy than the fully occupied states of Teflon. These partially occupied states split lower total energy before water adsorption and lead to ferromagnetic configuration ( Fig. 5e ). However, charge transfer between water molecule and dangling bonds transform the ferromagnetic configuration between dangling bonds into weak AFM configuration, as shown in Supplementary Fig. S4 . It is noted that the calculated adsorption energy (−0.48 eV) of water molecule to the end of the Teflon chain is close to the experimentally determined value of the activation energy 0.2 eV ( Supplementary Fig. S5 ). The relatively weak interaction between the C dangling bond and H 2 O is thus the reason that FM in Teflon tape can be recovered by annealing at an elevated temperatures in Ar after it is eliminated by steam annealing, as the subsequent annealing in Ar evaporates the attached water molecules. Room temperature FM in polyethylene If FM can be created in Teflon tape by simple stretching, heating and cutting, it is natural to ask whether ferromagnetic coupling can also be established in other polymers using these methods and whether this is a common phenomenon. To answer this question, we carried out similar experiments on two kinds of polyethylene (PE, -(CH 2 ) n -) sheets (pure high-density PE (HDPE) and low-density PE (LDPE) purchased form Sigma-Aldrich). Both HDPE and LDPE sheets were found to show room temperature FM after being cut under pure N 2 or Ar ( Table 1 ). However, when it is cut in air, the sample is nonmagnetic. In addition, FM was not observed after the sample is cut under 0.1% H 2 /Ar or 2.5% H 2 /Ar. These results may suggest that the C–H bond could be easily formed in PE. Once the FM is eliminated, further annealing under Ar at 50 and 80 °C (just below the melting temperature of ∼ 100 °C), does not lead to recovery of FM. Our first-principle calculations on PE indicate that the ferromagnetic ordering can be realized in the 2D network of C dangling bonds, similar to that of Teflon, and the ferromagnetic ordering collapses if these C dangling bonds are saturated by H ions. As FM in PE is unstable in air, mechanical stretching was not carried out on PE samples (HDPE and LDPE). In summary, room temperature FM has been observed in Teflon tape after mechanical stretching, cutting or annealing. The magnetic moments originate from C dangling bonds and FM is established through a relatively strong coupling between neighbouring C dangling bonds in the 2D network formed in the cross-section of broken Teflon, or its vicinity. After a Teflon tape is cut, a relatively uniform 2D ferromagnet appears in the cross-sectional plane, as the measured magnetization is very close to the expected magnetization if all Teflon chains across the plane are broken and a 2D network of C dangling bonds is formed in the cross-section. The FM in Teflon tape after mechanical stretching is not uniform, and it is likely due to exchange coupling between connected C dangling bonds, which form chains or concentrate on surfaces of strain-induced lateral voids. The FM can be eliminated when the Teflon tape is exposed to H 2 due to the formation of C–H bond or by adsorption of water molecules. However, the FM in the latter can be recovered through annealing while that in the former is permanently eliminated. Room temperature FM can also be realized in PE sheets by cutting under N 2 or Ar atmosphere, even though it is unstable in air, possibly due to formation of C–H bonds, suggesting that FM may be produced by simply stretching or cutting in all polymer systems. Our work explains the FM in polymers that may have been observed by many research groups worldwide, whereas the mechanism has not been understood. This work demonstrates the formation of a new type of ferromagnet—a 2D C dangling bond network in a polymeric material. By simply stretching or cutting a carbon-based material or a polymers/organic material, one can easily create a ferromagnetic structure. Our work has shown that C dangling bonds are relatively stable in Teflon. The adsorption and removal of water molecule can be explored to realize an on/off switching device. Furthermore, C dangling bond structures may be created through cleave engineering and protected by coating. This may lead to nano-magnetic designs in polymeric and molecular materials for various applications such as in spintronics devices. Sample preparation Teflon tape (high-purity polytetrafluoroethylene, -(CF 2 ) n ) was purchased from Sigma-Aldrich. Strips of Teflon tape with a typical length of 10 cm and a typical mass of 0.08 g were used in our experiments. For mechanical stretching, the Teflon strip was fixed on plastic rods and pulled slowly until it is broken. To avoid magnetic contamination, the Teflon tape was cut with a pair of ceramic scissors. The cut samples were immediately sealed in a plastic holder for magnetic characterization. Annealing was done in a tube furnace under a controlled atmosphere (pure N 2 , pure Ar, 20%O 2 /80%Ar 2.5%H 2 /97.5%Ar, 0.1%H 2 /Ar and water steam) for 2 h at a temperature in the range of 50–350 °C. Magnetic measurements were carried out within 10 min after the samples were undergone heat treatment. To confirm the FM in 2D network of C dangling bonds that may exist in other polymeric materials, we also examined LDPE and HDPEsheets (purchased from Sigma-Aldrich) after mechanical stretching or cutting. Structural characterization and magnetic measurements XRD, Raman spectroscopy and FTIR were used to characterize the structure of the Teflon tape. For the analysis of composition and possible magnetic impurities, we used EDS attached to a scanning electron microscopy system (Philips, XL-30), ICP (Optima 5300 DV ICP-OES), Time-of-flight SIMS (TOF-SIMS, ION TOF SIMS IV) and XPS (Kratos AXIS Ultra DLD) for the elemental analysis. In order to avoid charging due to the insulating behaviour of the tape, the tape is coated with a layer of 10-nm gold film for TOF-SIMS examination. The signal from gold was not taken into the consideration. In addition, an electron gun was used for charge compensation. Ga ions are used for the SIMS measurement with negative polarity. Similarly, in the XPS analysis, an electron gun was also used for the charge compensation. Teflon tape was flattened on the surface of glass substrate with conductive carbon and aluminium tape. In order to rule out the possibility of FM due to contamination, composition measurements were carried out before and after magnetic measurements. A superconducting quantum interference device (Quantum Design, MPMS XL-5) system was used for the magnetic characterization. Saturation magnetization is obtained by averaging the values of at least three samples. The ESR spectra were taken with a JEOL JES FA300 system (JEOL) with a microwave power of 0.1 mW and microwave frequency of 8.984 GHz. For the sample with highest saturation magnetization (after annealing at 150 °C as shown in Fig. 3a ), ESR measurements were taken at different temperatures in the range of 80 K (LN 2 ) and 300 K (room temperature). First-principles calculations First-principles calculations were performed using the VASP code [30] . The ultrasoft peusdo-potentials were used to model electron–ion interactions. Structure relaxation was carried out using the generalized gradient approximation (GGA) [31] for exchange-correlation function. Electronic properties (total energy, DOS, band structure) calculated using GGA were verified by hybrid functional available in the CRYSTAL code [32] . Results obtained using different functionals (B3LYP, SOGGAXC and PBE0) are consistent. All results presented are based on PBE0 except those given in Supplementary Table S3 , which were obtained using GGA. The k-space integration was done by summing over the Monkhorst-Pack [32] special points in the Brillouin zone. The Gaussian method, with a smearing width of 0.01 eV was used in determination of the Fermi level. The plane wave basis set was restricted by cutoff energy of 425 eV. A slab model was used to simulate the fractured surfaces and a 15 Å vacuum region was used to ensure that there is negligible interaction between surfaces in neighbouring cells. The forces acting on atoms are <0.05 eV Å −1 in the optimized structures. DOS calculations were performed using a hexagonal 4.7 Å×4.7 Å unit cell for each Teflon chain with k-spacing <0.02/Å. How to cite this article: Ma, Y. W. et al . Room temperature ferromagnetism in Teflon due to carbon dangling bonds. Nat. Commun. 3:727 doi: 10.1038/ncomms1689 (2012).